SCARECROW-LIKE15 interacts with HISTONE DEACETYLASE19 and is essential for repressing the seed maturation programme Epigenetic regulation of gene expression is critical for controlling embryonic properties during the embryo-to-seedling phase transition. Here we report that a HISTONE DEACETYLASE19 (HDA19)-associated regulator, SCARECROW-LIKE15 (SCL15), is essential for repressing the seed maturation programme in vegetative tissues. SCL15 is expressed in and GFP-tagged SCL15 predominantly localizes to, the vascular bundles particularly in the phloem companion cells and neighbouring specialized cells. Mutation of SCL15 leads to a global shift in gene expression in seedlings to a profile resembling late embryogenesis in seeds. In scl15 seedlings, many genes involved in seed maturation are markedly derepressed with concomitant accumulation of seed 12S globulin; this is correlated with elevated levels of histone acetylation at a subset of seed-specific loci. SCL15 physically interacts with HDA19 and direct targets of HDA19–SCL15 association are identified. These studies reveal that SCL15 acts as an HDA19-associated regulator to repress embryonic traits in seedlings. Seed development is an intricate process that begins with double fertilization followed by embryogenesis and seed maturation, the latter being characterized by the expression of embryonic traits such as accumulation of seed storage reserves [1] . The initiation of the seed maturation processes is mainly controlled by three B3 domain transcription factors, namely LEAFY COTYLEDON2 (LEC2), ABSCISIC ACID (ABA) INSENTITIVE3 (ABI3) and FUSCA3 (FUS3). These factors work in consort with the CCAAT-box binding factor (CBF) LEC1, ABA, auxin, gibberellin and sugar signalling [1] , [2] . Transition from the seed maturation to the vegetative phase is thought to be controlled by different mechanisms including environmental cues, hormonal signalling, metabolic changes and transcriptional regulation [3] , [4] , [5] . During seed germination and seedling establishment after release of seed dormancy, the seed maturation programme is repressed so that embryonic traits are not expressed in vegetative tissues. Chromatin modifications have been implicated in repressing embryonic traits during seed germination and vegetative growth. Inactivation of the bean ( Phaseolus vulgaris ) phaseolin ( phas ) gene in vegetative tissues is attributed to nucleosome positioning over its TATA regions [6] . Histone methylation and acetylation are associated with the chromatin remodelling and activation of the phas promoter [7] . The CHD3 chromatin remodelling factor PICKLE (PKL) acts in consort with gibberellic acid to ensure that embryonic traits are not expressed during germination [8] . Furthermore, PKL acts directly upon LEC1, LEC2 and FUS3 that are enriched for trimethylation of histone H3 lysine 27 (H3K27me3) [9] . Polycomb (PcG) group proteins play a key role in maintaining the epigenetic states of repressed genes via H3K27me3. The PcG repressive complex 2 (PRC2) is essential for controlling transition from the embryonic phase to the seedling stage by deposition of repressive H3K27me3 mark on seed maturation genes [10] . B3 domain transcription factors and seed maturation genes for 2S albumin, 12S globulin and oleosin possess H3K27me3 marks in vegetative tissues [11] . Derepression of FUS3 in leaves is directly associated with the PcG protein MEDEA [12] , and repression of LEC2 during vegetative growth is regulated by a Repressive LEC2 Element ( RLE ) that is essential for the deposition of H3K27me3 marks [13] . The VP1/ABI3-LIKE (VAL) B3 proteins VAL1, VAL2 and VAL3 (also known as HSI2, HSL1 and HSL2, respectively) [14] are essential for the repression of sugar-inducible embryonic traits in seedlings [14] , [15] , [16] . The PHD-L domain of VAL1 was found to repress seed maturation genes through, at least in part, regulation of histone methylation on target genes [17] . Recently, the CW-Zf domain of VAL2 was demonstrated to interact with HISTONE DEACETYLASE19 (HDA19) [18] and VAL proteins act together with a member of the PRC1, AtBMI1, to initiate the embryo-to-seedling phase transition in Arabidopsis [19] . A BRAHMA-containing SNF2 complex in the SWI/SNF family was shown to repress seed genes in Arabidopsis leaves [20] . Mutations affecting SDG8 (SET DOMAIN GROUP 8) caused ectopic expression of a subset of seed maturation genes in leaves [21] . Overexpression of miR166 targets, the type III homeodomain-leucine zipper genes PHABULOSA ( PHB ) and PHAVOLUTA ( PHV ), activated embryonic genes in vegetative tissues [22] . In addition, a trihelix DNA-binding factor ARABIDOPSIS6b-INTERACTING PROTEIN1-LIKE1 (ASIL1) was shown to directly target the GT cis -element (5’-GTGATT) of At2S3 in vitro and is essential for the repression of the seed regulatory network in Arabidopsis seedlings [23] . Histone acetyltransferases and histone deacetylases (HDACs) play a critical role in the regulation of gene expression and they are commonly associated with other transcriptional regulators to form multi-subunit protein complexes for specific cellular functions [24] . The reversible acetylation and deacetylation of histones are generally accompanied with the activation and silencing of gene expression, respectively [24] . HDA19 was shown to have HDAC activity in vitro and to form a multiprotein complex for the repression of gene expression [25] . HDAC activity is thought to be important for the repression of certain seed-specific genes [26] . More specifically, HDA6 and HDA19 contribute redundantly to the repression of embryonic properties after germination [18] , [27] , although the underlying mechanism remains unclear. Here, using a yeast two-hybrid system, we identify SCARECROW (SCR)-LIKE15 (SCL15) as being associated with HDA19. The interaction of SCL15 with HDA19 is confirmed using glutathione S -transferase (GST) pull-down, bimolecular fluorescence complementation (BiFC), and co-immunoprecipitation (co-IP) assays. Promoter activity analysis and green fluorescent protein (GFP)-tagged protein localization show that SCL15 is predominantly expressed in the phloem companion cells (CCs), as well as in specialized cells that are adjacent to the CCs. We demonstrate that SCL15 is required for the repression of a large subset of seed maturation genes and provide evidence that ectopic expression of embryonic genes in scl15-1 seedlings correlates with the histone H3 hyperacetylation of chromatin at seed-specific loci. Moreover, some of these loci are identified as direct targets of HDA19–SCL15 association. These findings suggest that SCL15 acts as part of an HDA19-associated complex to repress the expression of embryonic genes in seedlings and is involved in the regulation of embryo-to-seedling phase transition. SCL15 is a nuclear GRAS protein To identify proteins that interact with HDA19, the full-length Arabidopsis HDA19 fused to the yeast GAL4 DNA-binding domain (GAL4 DB) was used as bait to screen an Arabidopsis seedling cDNA library. A total of 1.6 × 10 6 yeast transformants were screened yielding nine positive clones. One of these clones encoded SCL15 (At4g36710), which is also designated as AtHAM4 based on its genetic interaction with two Petunia HAIRY MERISTEM (HAM) homologues AtHAM1 and AtHAM2 (ref. 28 ). Comparison of deduced amino-acid sequences showed that SCL15 and the HAM homologues AtHAM1, AtHAM2 and AtHAM3 were fairly divergent, showing only 28–31% identity at the amino-acid level ( Supplementary Fig. 1 ). SCL15 shared 86% amino-acid identity with BnSCL1, an auxin responsive HDA19-interacting protein in Brassica napus [29] and a member of the plant-specific GRAS (GIBBERELLIN ACID INSENSITIVE (GAI), REPRESSOR OF GIBBERELLIC ACID INSENSITIVE3 (RGA) and SCR) [30] protein family. Phylogenetic analysis of all the Arabidopsis GRAS proteins confirmed their relationships ( Supplementary Fig. 2 ) [31] . Most GRAS domain proteins identified so far are nuclear proteins and SCL15 was shown to be mainly nuclear localized [31] . To confirm the nuclear localization of SCL15, a transient expression assay was conducted in tobacco epidermal cells with a soluble-modified red-shifted green fluorescent protein (smRS-GFP) translational fusion. The SCL15-smRS-GFP was localized only in the nuclei ( Supplementary Fig. 3 ), indicating that SCL15 is a nuclear-restricted GRAS protein. SCL15 physically associates with HDA19 To corroborate the physical association between SCL15 and HDA19 detected in the yeast two-hybrid system, three kinds of assays were conducted. First, in vitro GST pull-down affinity assays were performed. [ 35 S]methionine-labelled SCL15 protein was tested for its ability to interact with recombinant GST–HDA19 fusion protein. SCL15 bound to GST-HDA19 fusion protein, but not to GST alone ( Fig. 1a ). Second, BiFC assays in Arabidopsis protoplasts were carried out. SCL15 was fused to the N-terminal yellow fluorescent protein (YFP) fragment and HDA19 was fused to the C-terminal YFP fragment. A yellow fluorescent signal was observed when SCL15-N-YFP was co-delivered into protoplasts with HDA19-C-YFP ( Fig. 1b and Supplementary Fig. 4 ). Third, a co-IP experiment was performed using nuclear protein extracts from roots of T3 homozygous SCL15pro::SCL15-sGFP transgenic plants that were in an scl15-1 background and had been used for the complementation assays. This assay showed that HDA19 co-precipitated with SCL15-sGFP ( Fig. 1c ). These results provide good evidence that SCL15 physically interacts with HDA19 in the nuclei of Arabidopsis cells. 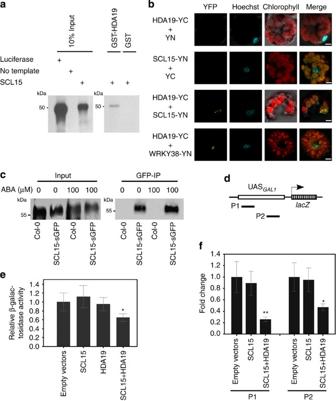Figure 1: Physical interaction of SCL15 with HDA19. (a) GST pull-down assay showing interaction of SCL15 with HDA19in vitro. SCL15 was expressed and radiolabelled usingin vitrotranscription/translation reactions. The translation product (input) was incubated with GST-HDA19 fusion or GST alone. (b) BiFC assay displaying SCL15 interaction with HDA19 in the nucleus ofArabidopsisprotoplasts. Co-expression of SCL15-YN or HDA19-YC with empty vector YC or YN was used as a negative control and co-expression of HDA19-YC and WRKY38-YN served as a positive control for the BiFC assay. Scale bars, 5 μm. (c) Co-IP assay inArabidopsisseedlings showing co-precipitation of HDA19 with SCL15-sGFP. Nuclear extracts (Input) from wild-type Col-0 or homozygous transgenic plants stably expressingSCL15pro::SCL15-sGFPtreated with or without ABA were immunoprecipitated with a polyclonal anti-GFP antibody (GFP-IP) followed by western blot analysis with polyclonal anti-HDA19 antibodies. (d) Schematic diagram of the yeastGAL1procontaining Gal4-responsive Upstream Activating Sequences UASGAL1and the regions examined after ChIP. (e) Co-expression ofHDA19andSCL15-GAL4BDin aGAL4UAS-GAL1pro::LacZyeast reporter line exhibits reduced level ofLacZ expression when compared with SCL15-GAL4BD alone or empty vectors. Expression data represent the mean (±s.d.) of three biological replicates (Student’st-test, *P<0.05). (f) Levels of H3K9ac in the P1 and P2 regions ofGAL1pro. The fold enrichment of SCL15+HDA19 over SCL15 only is shown and the values are means±s.d. from three biological replicates (Student’st-test, *P<0.05, **P<0.01). Figure 1: Physical interaction of SCL15 with HDA19. ( a ) GST pull-down assay showing interaction of SCL15 with HDA19 in vitro . SCL15 was expressed and radiolabelled using in vitro transcription/translation reactions. The translation product (input) was incubated with GST-HDA19 fusion or GST alone. ( b ) BiFC assay displaying SCL15 interaction with HDA19 in the nucleus of Arabidopsis protoplasts. Co-expression of SCL15-YN or HDA19-YC with empty vector YC or YN was used as a negative control and co-expression of HDA19-YC and WRKY38-YN served as a positive control for the BiFC assay. Scale bars, 5 μm. ( c ) Co-IP assay in Arabidopsis seedlings showing co-precipitation of HDA19 with SCL15-sGFP. Nuclear extracts (Input) from wild-type Col-0 or homozygous transgenic plants stably expressing SCL15pro::SCL15-sGFP treated with or without ABA were immunoprecipitated with a polyclonal anti-GFP antibody (GFP-IP) followed by western blot analysis with polyclonal anti-HDA19 antibodies. ( d ) Schematic diagram of the yeast GAL1pro containing Gal4-responsive Upstream Activating Sequences UAS GAL1 and the regions examined after ChIP. ( e ) Co-expression of HDA19 and SCL15-GAL4BD in a GAL4UAS-GAL1pro::LacZ yeast reporter line exhibits reduced level of Lac Z expression when compared with SCL15-GAL4BD alone or empty vectors. Expression data represent the mean (±s.d.) of three biological replicates (Student’s t -test, * P <0.05). ( f ) Levels of H3K9ac in the P1 and P2 regions of GAL1pro . The fold enrichment of SCL15+HDA19 over SCL15 only is shown and the values are means±s.d. from three biological replicates (Student’s t -test, * P <0.05, ** P <0.01). Full size image To test whether SCL15–HDA19 interaction affects the histone acetylation status at a target promoter, a SCL15-GAL4DB fusion was used to co-transform a yeast line with pGAL1-HDA19 . The yeast strain ( GAL4UAS-GAL1pro::lacZ ) harbours an integrated lac Z gene under the control of the GAL1 promoter and is regulated by distinct GAL4-responsive Upstream Activating Sequences (UAS GAL1 ; Fig. 1d ). Co-transformation of SCL15-GAL4DB with p426GAL1-HDA19 resulted in reduced β-galactosidase activity when compared with SCL15-GAL4BD alone or empty vectors ( Fig. 1e ). Chromatin immunoprecipitation (ChIP) assays were then conducted to investigate whether co-expression of SCL15 with HDA19 led to changes in the histone acetylation state at the GAL1 promoter. The histone H3K9 acetylation (H3K9ac) levels around the UAS GAL1 sites were significantly reduced when both SCL15-GAL4DB and p426GAL1-HDA19 were expressed compared with SCL15-GAL4DB or the vectors alone ( Fig. 1f ). This suggests that SCL15 recruits HDA19 to the target promoter via a gene-specific DNA-binding domain to decrease the local histone acetylation levels. Phenotypic characterization of scl15 mutants For the functional analysis of SCL15 in planta , we obtained two independent T-DNA insertion lines for the SCL15 gene, namely SALK_110871 ( scl15-1 , also referred to as Atham4-1 (ref. 28 ), and GK292A11 ( scl15-2 ). Based on the available description of the two T-DNA insertion lines ( http://www.arabidopsis.org and http://www.gabi-kat.de ), the T-DNA insertion site was located in the coding region of SCL15 gene, 1,004 and 1,064 bp downstream of the translation start site, respectively ( Fig. 2a ). Both of the T-DNA insertions were located in the region encoding the PFYRE domain of SCL15 protein. No transcript was detected in the homozygous mutant plants using reverse transcription (RT)–PCR analysis with primers that either spanned the T-DNA insertions or were downstream of the insertion sites. However, RT–PCR products were amplified when using primers located upstream of the T-DNA insertions ( Fig. 2b ). This result indicates that transcription of the full-length SCL15 in the mutant plants is disrupted by the T-DNA insertion, but that scl15-1 and scl15-2 could be hypomorphic rather than null mutations. 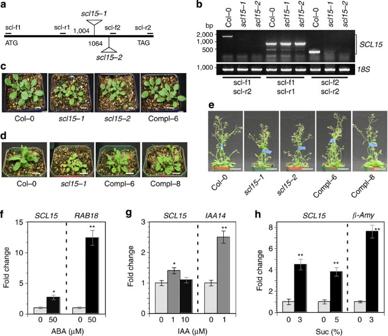Figure 2: Effects ofSCL15mutation on plant growth and response to ABA and sugar. (a) Schematic representation of the T-DNA insertion alleles of SALK_110871 (scl15-1)and GK292A11 (scl15-2) inArabidopsis. Numbers indicate positions of T-DNA insertions with respect to the start of translation. The positions of PCR primers for RT–PCR analysis are also indicated. (b) RT–PCR analysis of total RNA from leaves of wild-type Col-0 and homozygousscl15-1andscl15-2plants with several primer pairs. (c) Phenotypes of 15-day-old wild-type, homozygousscl15mutants and a complementedSCL15pro::SCL15-GFPline (Compl-6) plantlets. Scale bar, 1 cm. (d) Wild-type,scl15mutant and complemented lines (Compl-6 and Compl-8) at 21 days of growth. Scale bar, 2 cm. (e) Wild-type,scl15mutants and complementedSCL15pro::SCL15-GFPlines at 32 days of growth. Scale bar, 5 cm. (f)SCL15expression 2 days after ABA treatment, (g) 1 h after IAA treatment and (h) 1 h after sucrose treatment.RAB18,β-AmyandIAA14served as controls to validate the ABA, sugar and auxin responses, respectively. Expression data represent the mean (±s.d.) of three biological replicates (Student’st-test, *P<0.05; **P<0.01). Figure 2: Effects of SCL15 mutation on plant growth and response to ABA and sugar. ( a ) Schematic representation of the T-DNA insertion alleles of SALK_110871 ( scl15-1) and GK292A11 ( scl15-2 ) in Arabidopsis . Numbers indicate positions of T-DNA insertions with respect to the start of translation. The positions of PCR primers for RT–PCR analysis are also indicated. ( b ) RT–PCR analysis of total RNA from leaves of wild-type Col-0 and homozygous scl15-1 and scl15-2 plants with several primer pairs. ( c ) Phenotypes of 15-day-old wild-type, homozygous scl15 mutants and a complemented SCL15pro::SCL15-GFP line (Compl-6) plantlets. Scale bar, 1 cm. ( d ) Wild-type, scl15 mutant and complemented lines (Compl-6 and Compl-8) at 21 days of growth. Scale bar, 2 cm. ( e ) Wild-type, scl15 mutants and complemented SCL15pro::SCL15-GFP lines at 32 days of growth. Scale bar, 5 cm. ( f ) SCL15 expression 2 days after ABA treatment, ( g ) 1 h after IAA treatment and ( h ) 1 h after sucrose treatment. RAB18 , β-Amy and IAA14 served as controls to validate the ABA, sugar and auxin responses, respectively. Expression data represent the mean (±s.d.) of three biological replicates (Student’s t -test, * P <0.05; ** P <0.01). Full size image There were no significant abnormalities in plant growth in scl15-1 and scl15-2 plants, as previously described [28] , [31] , although they exhibited differences in vegetative growth and development from the wild type before the mid-stage of plant development. The mutant seedlings were smaller than those of the wild type and flowering was delayed by 2 to 3 days in long days when compared with the wild type. The mean rosette leaf numbers of the scl15 and wild-type plants were 12.8±0.6 and 13.9±0.8 (±indicates standard deviation, n =10), respectively ( Fig. 2c,d ). The scl15 adult plants at the 32-day-old stage were still shorter (24.9±0.7 cm) than the wild type (30.8±0.8 cm; Student’s t -test, P <0.01; Fig. 2e ), but subsequently caught up and had a life cycle from germination to mature seeds of about the same duration as wild-type plants. To confirm the phenotypes exhibited in scl15 mutant plants, complementation assays were conducted. The SCL15 genomic sequence fused to sGFP ( SCL15pro::SCL15-sGFP ) was used to transform scl15-1 mutant plants. Five independent transgenic lines displaying a 3:1 segregation ratio in T2 populations were selected and two of the T3 homozygous lines, Compl-6 and Compl-8, were chosen for the complementation assays. The SCL15-sGFP fusion protein was able to complement the scl15-1 mutant phenotypes ( Fig. 2c–e ). There was no difference between the phenotypes of complemented lines and wild-type plants in terms of seedling establishment, flowering and plant growth, indicating that SCL15-sGFP fusion protein is functional. ABA, auxin, sugar and GA are important cues that guide seed maturation and the transition to seed germination [1] , [3] . The effect of ABA, sugar and auxin on SCL15 expression was tested. The level of SCL15 transcript increased substantially in response to ABA and sucrose, whereas SCL15 expression was only moderately altered by auxin treatment ( Fig. 2f–h ). SCL15 is predominantly expressed in phloem CCs The specific expression of SCL15 in vascular tissues, particularly in the root phloem system and chalazal seed coat has been suggested from information in in silico databases, the BAR Arabidopsis eFP browser ( http://bar.utoronto.ca/efp/cgi-bin/efpWeb.cgi ) and Genevestigator ( https://www.genevestigator.com/gv/plant.jsp ; Supplementary Fig. 5 ). To confirm the expression pattern, we analysed SCL15 promoter β-glucuronidase (GUS) activity and SCL15-GFP protein localization. The SCL15 promoter- GUS construct was generated by fusing the 2.3-kb fragment directly upstream of the SCL15 start codon to the GUS reporter gene and six independent transformants were analysed. In T1 transgenic Arabidopsis plants, strong GUS staining was observed in the vascular tissues of cotyledons, leaves, stamen filaments and primary and lateral roots ( Fig. 3a–g ). During seed development, SCL15pro::GUS expression was not detected in the embryo ( Fig. 3h,i ), whereas a strong GUS signal was found in the funiculi and chalazal regions of ovules and mature seeds ( Fig. 3j–l ), as well as the vasculature of silique walls ( Fig. 3m ). 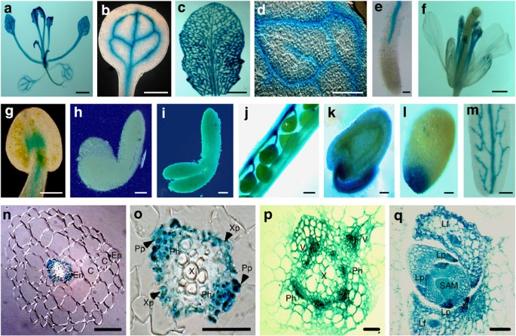Figure 3: Tissue-specific expression ofSCL15. (a–e) GUS activity was assayed in a 28-day-oldSCL15pro::GUSseedling. (a) Whole seedling. (b) Cotyledon. (c) Fully expanded leaf. (d) Portion of leaf surface showing the GUS activity in leaf veins. (e) Root tip. (f,g) GUS staining in floral organs. (f) Flower. (g) Anther. (h–m)pSCL15::GUSexpression in developing seeds. (h) Ovules in silique at 4 days post-anthesis (DPA). (i) Silique wall at 8 DPA. (j) Early bending stage embryo. (k) Late bending stage embryo. (l) Ovule at 4 DPA. (m) Mature seed. (n) Transverse section of a root tip showing that GUS activity is exclusively restricted to the vascular bundle. (o) Magnified vascular bundle showing that GUS expression is primarily localized at the abaxial side of the vascular bundle. (p) Transverse section of a stem. (q) Longitudinal section of a shoot apex showing GUS activity in developing leaf primordia and vascular tissues of older leaf primordia. C, cortex; En, endodermis; Ep, epidermis; Lf, leaf; Lp, leaf primordia; Ph, phloem; Pp, phloem-pole pericycle; SAM, shoot apical meristem; V, vascular tissue; X, xylem; Xp, xylem-pole pericycle. Scale bars, 2 nm ina–c, 200 μm indandf, 100 μm ine,gandq, 50 μm inh,i,k,landn, 150 μm injandm, 20 μm inoandp. Figure 3: Tissue-specific expression of SCL15 . ( a – e ) GUS activity was assayed in a 28-day-old SCL15pro::GUS seedling. ( a ) Whole seedling. ( b ) Cotyledon. ( c ) Fully expanded leaf. ( d ) Portion of leaf surface showing the GUS activity in leaf veins. ( e ) Root tip. ( f , g ) GUS staining in floral organs. ( f ) Flower. ( g ) Anther. ( h – m ) pSCL15::GUS expression in developing seeds. ( h ) Ovules in silique at 4 days post-anthesis (DPA). ( i ) Silique wall at 8 DPA. ( j ) Early bending stage embryo. ( k ) Late bending stage embryo. ( l ) Ovule at 4 DPA. ( m ) Mature seed. ( n ) Transverse section of a root tip showing that GUS activity is exclusively restricted to the vascular bundle. ( o ) Magnified vascular bundle showing that GUS expression is primarily localized at the abaxial side of the vascular bundle. ( p ) Transverse section of a stem. ( q ) Longitudinal section of a shoot apex showing GUS activity in developing leaf primordia and vascular tissues of older leaf primordia. C, cortex; En, endodermis; Ep, epidermis; Lf, leaf; Lp, leaf primordia; Ph, phloem; Pp, phloem-pole pericycle; SAM, shoot apical meristem; V, vascular tissue; X, xylem; Xp, xylem-pole pericycle. Scale bars, 2 nm in a – c , 200 μm in d and f , 100 μm in e , g and q , 50 μm in h , i , k , l and n , 150 μm in j and m , 20 μm in o and p . Full size image A more detailed analysis of SCL15pro::GUS expression pattern was performed using a dissecting microscope. GUS activity was exclusively restricted to the vascular bundles in mature root and a stronger signal was detected on the abaxial (phloem system) sides of root and stem vascular bundles, whereas no GUS activity was found in the adaxial xylem vessels ( Fig. 3n–p ). In vegetative apices, GUS activity was observed in the newly formed leaf primordia and the vasculatures of older leaf primordia ( Fig. 3q ). SCL15 localization was examined in vascular tissues of the scl15-1 mutant expressing SCL15pro::SCL15-sGFP that had been used for the complementation assays. The GFP signal occurred in the phloem CCs as well as in the neighbouring tissues. In leaf petiole, the signal was apparent in the CCs and neighbouring bundle sheath (BS) cells ( Fig. 4a,b ). At the root tip, SCL15-sGFP fluorescence was predominantly localized in protophloem sieve elements and neighbouring phloem-pole pericycle cells (Pp; Fig. 4c,d ). In mature roots, the signal was restricted to the nuclei of metaphloem CCs and the Pp cells ( Fig. 4e,f ). In developing seeds, SCL15pro::SCL15-sGFP was expressed in the CCs of chalazal ends of the ovule funiculi, a tissue that connects the ovule to the ovary wall. Interestingly, a strong GFP signal was also present in the placentochalaza, a region that is in close proximity to the CCs at the base of the funiculus vasculature ( Fig. 4g–j ) and is thought to function as a nutrient unloading zone, particularly for the export of amino acids [32] , [33] . 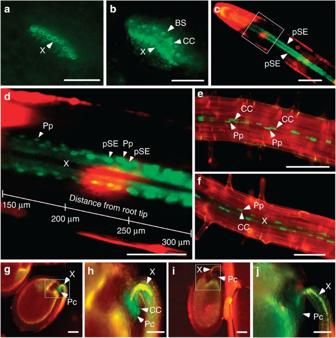Figure 4: Cell-specific localization of SCL15-sGFP inArabidopsis. (a) Leaf petiole cross-sections of wild-typeArabidopsis. (b) Leaf petiole cross-sections ofSCL15pro::SCL15-sGFPtransgenic plants showing localization of SCL15-GFP fusion in companion cells (CCs) and neighbouring bundle sheath (BS) cells. (c) Primary root tip from a 3-day-oldSCL15pro::SCL15-sGFPseedling displaying GFP localization in protophloem sieve element (pSE). (d) The proximal meristem region boxed incis magnified indshowing GFP fluorescence is present in pSE as well as in phloem-pole pericycle (Pp) cells. (e) SCL15pro::SCL15-sGFP localization in CCs and neighbouring Pp cells of the primary root. One phloem pole is shown when viewed perpendicular to the xylem axis. (f) Two phloem poles are shown when viewed perpendicular to the axis of two phloem poles. (g) Developing seed from aSCL15pro::SCL15-GFPplant showing GFP signal in CCs and neighbouring Pc cells. (h) The chalazal seed coat region boxed ingis magnified. (i) Developing seed from a wild-type Col-0 plant. (j) The chalazal seed coat region boxed iniis magnified. Pc, placentochalaza; Ps, pigment strand; X, xylem. Scale bars, 100 μm ina–c,e–gandi, and 50 μm ind,handj. Figure 4: Cell-specific localization of SCL15-sGFP in Arabidopsis . ( a ) Leaf petiole cross-sections of wild-type Arabidopsis . ( b ) Leaf petiole cross-sections of SCL15pro::SCL15-sGFP transgenic plants showing localization of SCL15-GFP fusion in companion cells (CCs) and neighbouring bundle sheath (BS) cells. ( c ) Primary root tip from a 3-day-old SCL15pro::SCL15-sGFP seedling displaying GFP localization in protophloem sieve element (pSE). ( d ) The proximal meristem region boxed in c is magnified in d showing GFP fluorescence is present in pSE as well as in phloem-pole pericycle (Pp) cells. ( e ) SCL15pro::SCL15-sGFP localization in CCs and neighbouring Pp cells of the primary root. One phloem pole is shown when viewed perpendicular to the xylem axis. ( f ) Two phloem poles are shown when viewed perpendicular to the axis of two phloem poles. ( g ) Developing seed from a SCL15pro::SCL15-GFP plant showing GFP signal in CCs and neighbouring Pc cells. ( h ) The chalazal seed coat region boxed in g is magnified. ( i ) Developing seed from a wild-type Col-0 plant. ( j ) The chalazal seed coat region boxed in i is magnified. Pc, placentochalaza; Ps, pigment strand; X, xylem. Scale bars, 100 μm in a–c , e – g and i , and 50 μm in d , h and j . Full size image SCL15 represses seed maturation genes in vegetative tissue Microarray analysis on scl15-1 and wild-type seedlings was performed to obtain global changes in gene expression caused by SCL15 mutation. Global gene expression patterns in wild-type and the scl15-1 mutant seedlings were profoundly different, such that 606 genes were at least twofold upregulated and 363 genes were more than twofold downregulated in the mutant relative to the wild type (Student’s t -test ( P ≤0.05) from three biological replicates with a Benjamini-Hochberg false discovery rate of 0.05; Supplementary Data 1 and 2 ). To evaluate the upregulated genes, BiNGO analysis was used to assign gene ontology (GO) categories to the 209 genes that showed more than threefold higher expression in the mutant seedlings [34] . Most of the over-represented GO categories in the classification system biological function related to reproduction with two distinct subcategories: stress response and seed development ( Fig. 5 and Supplementary Fig. 6 ). The seed development group of genes related to those that are fundamental for various aspects of seed maturation and seed filling, namely genes encoding seed storage proteins (SSPs) and oleosins. The stress response group of genes were linked with environmental stress responses and hormone signalling, such as dehydration, cold stress and ABA signalling. However, a closer analysis of the corresponding genes revealed that most of them are also involved in embryogenesis and seed maturation. Besides reproduction and response to stimuli, a few additional small categories were also over-represented, including genes involved in lipid localization and vascular protein processing. These results suggest that SCL15 represses a large subset of seed maturation genes during the embryonic phase to seedling transition and during seedling establishment. 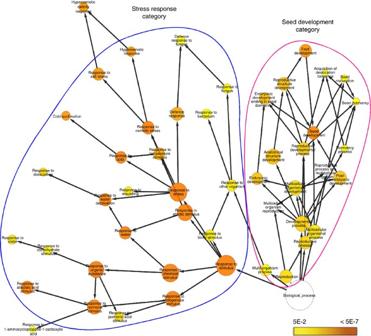Figure 5: Over-represented gene ontology (GO) categories among genes upregulated inscl15mutant seedlings. BiNGO analysis representing over-represented categories of the ontology Biological Process among the genes that are more than threefold (Student’st-test (P≤0.05) from three biological replicates with a Benjamini-Hochberg false discovery rate of 0.05) upregulated in thescl15-1mutant plants compared with the wild type. The two most over-represented GO categories ‘seed development’ and ‘stress response’ are shown. Coloured nodes ranging from yellow to dark orange represent the levels of significance of the over-represented GO terms withPvalues from 5E-2 to 5E-7 (Hypergeometric test and a Benjamini–HochbergP-value correction for multiple comparisons34,63). Figure 5: Over-represented gene ontology (GO) categories among genes upregulated in scl15 mutant seedlings. BiNGO analysis representing over-represented categories of the ontology Biological Process among the genes that are more than threefold (Student’s t -test ( P ≤0.05) from three biological replicates with a Benjamini-Hochberg false discovery rate of 0.05) upregulated in the scl15-1 mutant plants compared with the wild type. The two most over-represented GO categories ‘seed development’ and ‘stress response’ are shown. Coloured nodes ranging from yellow to dark orange represent the levels of significance of the over-represented GO terms with P values from 5E-2 to 5E-7 (Hypergeometric test and a Benjamini–Hochberg P -value correction for multiple comparisons [34] , [63] ). Full size image The DNA microarray results for embryonic genes that were markedly upregulated in scl15 mutant seedlings were validated using real-time RT–PCR. The tested genes are important in regulating initiation of the seed maturation programme ( LEC1 and ABI3 ), seed reserve trafficking and processing (vacuolar processing enzymes ( VPEs) , tonoplast intrinsic protein ( α-TIP ) and reticulon family gene ( RTNLB13 )) and accumulation ( CRA1 , CRU3 and Oleo2 ) [35] . Consistent with the microarray data, all of the genes noted above were upregulated in the mutant seedlings. Several were more than 20-fold upregulated, which included a seed-specific LEA (At4g21020) gene, RTNLB13 and CRA1 ( Fig. 6a , Supplementary Data 1 and Supplementary Table 1 ). Moreover, the expression of these seed maturation genes in scl15-1 seedlings expressing SCL15pro::SCL15-sGFP did not differ from wild-type plants ( Fig. 6b ). These results demonstrate that the ectopic expression of a subset of embryonic genes in seedlings is attributable to a defect in SCL15 expression and suggest that derepression of seed maturation genes in scl15 seedlings is mediated by upstream regulators in a manner analogous to that occurring in developing wild-type seeds. 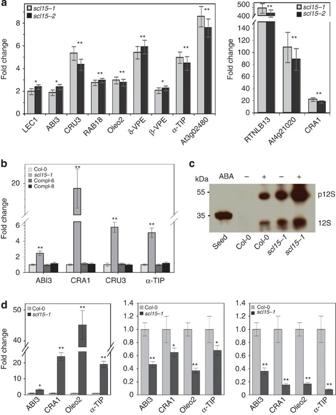Figure 6: Embryonic genes are ectopically expressed inscl15vegetative tissues. (a) Ectopic expression of seed maturation genes inscl15mutant seedlings. (b) Derepression of embryonic genes inscl15-1seedlings is restored to the wild-type levels by complementation withSCL15pro::SCL15-sGFP(Compl-6 and −8). (c) Immunoblot analysis with monoclonal anti-CRA1 antibody showing that accumulation of proglobulin (p12S) and 12S globulin species inscl15-1seedlings is increased by treatment with 50 μM ABA for 2 days. (d) Expression of seed maturation genes in siliques at the embryo morphogenesis stage (left), the mature (middle) and post-mature stages of embryo development (right). RNA levels are relative to the wild type (onefold). Results represent the mean (±s.d.) of three biological replicates (Student’st-test, *P<0.05; **P<0.01). Figure 6: Embryonic genes are ectopically expressed in scl15 vegetative tissues. ( a ) Ectopic expression of seed maturation genes in scl15 mutant seedlings. ( b ) Derepression of embryonic genes in scl15-1 seedlings is restored to the wild-type levels by complementation with SCL15pro::SCL15-sGFP (Compl-6 and −8). ( c ) Immunoblot analysis with monoclonal anti-CRA1 antibody showing that accumulation of proglobulin (p12S) and 12S globulin species in scl15-1 seedlings is increased by treatment with 50 μM ABA for 2 days. ( d ) Expression of seed maturation genes in siliques at the embryo morphogenesis stage (left), the mature (middle) and post-mature stages of embryo development (right). RNA levels are relative to the wild type (onefold). Results represent the mean (±s.d.) of three biological replicates (Student’s t -test, * P <0.05; ** P <0.01). Full size image To further investigate the extent to which the seed maturation prapram was derepressed in the mutant seedlings, we analysed scl15-1 for the presence of seed storage 12S globulins. Immunoblot analysis was conducted using monoclonal anti-CRA1 antibody against proteins extracted from 2-week-old seedlings. As shown in Fig. 6c , an unprocessed ∼ 55-kDa proglobulin (p12S) as well as 12S globulin species accumulated in untreated scl15-1 seedlings and accumulation of these proteins was increased after treatment with ABA. Globulins were not observed in untreated wild-type seedlings; however, accumulation of these proteins was detected after ABA treatment, although at much lower levels when compared with the ABA-treated scl15-1 seedlings ( Fig. 6c ). These findings indicates that in vegetative tissues ABA contributes to the derepression of genes encoding seed storage proteins. SCL15 was strongly expressed in the vascular tissues of silique walls, funiculi and chalazal regions of ovules and developing seeds ( Figs 3 and 4 ). Therefore, the expression of various seed maturation genes was examined, including ABI3 , α–TIP , CRA1 and Oleo2 , in developing siliques corresponding to embryo morphogenesis (5 days post-anthesis (DPA)), mature (10 DPA) and post-mature (16 DPA) stages of embryo development [32] . Seeds were matured and completely dry after 17 DPA. All seed maturation genes tested in siliques of scl15-1 mutant at 5 DPA were significantly upregulated, showing similar expression levels to that in seedlings. Heart to linear stage (5 DPA) of seed development is specialized in cellularization and tissue type differentiation before storage reserve accumulation [32] . However, transcripts of these genes were downregulated at the mature stage of embryo development and even further repressed at the post-mature stage compared with the wild type ( Fig. 6d ). HDA19–SCL15 association directly targets embryonic genes HDA19 is capable of forming a multiprotein complex for the repression of gene expression via histone deacetylation [25] and is involved in the repression of many seed maturation genes in Arabidopsis seedlings by reducing H3K14ac levels [18] . ChIP assay was performed to determine whether scl15-1 mutation affected histone acetylation at seed-specific loci that were derepressed in mutant seedlings. Increased acetyl H3K9K14 (H3K9K14ac) levels were found at the translational start regions and/or the proximal promoter regions in a subset of seed maturation genes in scl15-1 seedlings ( Fig. 7a,b ). These changes in histone acetylation state at the proximal promoter regions for derepressed seed genes in scl15-1 seedlings were restored to the wild-type levels in the presence of SCL15pro::SCL15-sGFP (Compl-6; Fig. 7c ). Histone H4 acetylation levels for ABI3 , CRA1 , CRU3 , AtEM6 and RAB18 were also elevated in the scl15-1 mutant ( Supplementary Fig. 7 ); however, H3 and H4 acetylation levels for LEC1 in the mutant were similar to those in the wild type ( Fig. 7a,b ). These results indicate that the ectopic expression of many embryonic genes in scl15-1 mutant seedlings was due, at least in part, to increased histone acetylation levels. 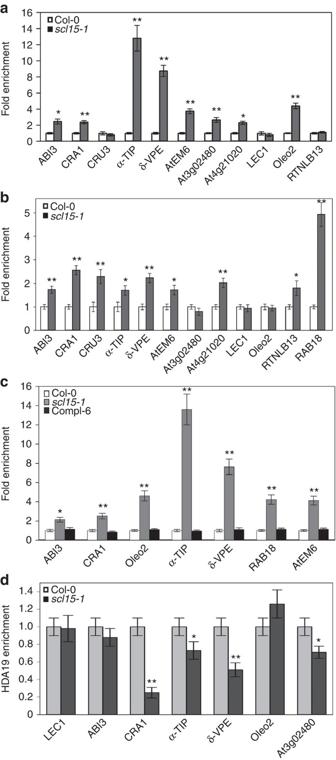Figure 7: ChIP analysis determines histone acetylation state at seed-specific loci. (a) H3K9K14ac levels at the proximal promoter regions and (b) the ATG regions of seed maturation genes in wild-type (Col-0) andscl15-1mutant seedlings. (c) H3K9K14ac levels for seed maturation genes in wild type, thescl15-1mutant and a homozygous complemented line stably expressingSCL15pro::SCL15-sGFP(Compl-6). (d)In vivodirect association of HDA19 with seed maturation genes in wild-type and thescl15-1mutant seedlings as determined by ChIP-qPCR assays with anti-HDA19 antibodies. The values obtained were normalized withACT7and the relative enrichment of HDA19 binding in wild type relative to thescl15-1and/or Compl-6 is shown as the mean±s.d. of three independent experiments (Student’st-test, *P<0.05, **P<0.01). Figure 7: ChIP analysis determines histone acetylation state at seed-specific loci. ( a ) H3K9K14ac levels at the proximal promoter regions and ( b ) the ATG regions of seed maturation genes in wild-type (Col-0) and scl15-1 mutant seedlings. ( c ) H3K9K14ac levels for seed maturation genes in wild type, the scl15-1 mutant and a homozygous complemented line stably expressing SCL15pro::SCL15-sGFP (Compl-6). ( d ) In vivo direct association of HDA19 with seed maturation genes in wild-type and the scl15-1 mutant seedlings as determined by ChIP-qPCR assays with anti-HDA19 antibodies. The values obtained were normalized with ACT7 and the relative enrichment of HDA19 binding in wild type relative to the scl15-1 and/or Compl-6 is shown as the mean±s.d. of three independent experiments (Student’s t -test, * P <0.05, ** P <0.01). Full size image To verify whether HDA19-SCL15 association plays a direct role in the repression of embryonic genes in seedlings, ChIP assays using anti-HDA19 antibodies were performed in wild-type and scl15-1 seedlings. The LEC1 gene was used as a negative control because it was derepressed without detectable changes in H3 and H4 acetylation levels in scl15-1 seedlings. Six embryonic genes encoding SSPs, oleosins and seed reserve trafficking proteins that were markedly derepressed ( Fig. 6 ) and displayed a dramatic increase in histone acetylation in scl15-1 seedlings ( Fig. 7 ) were examined. HDA19 was significantly enriched in the promoter regions of four genes, including the 12S globulin gene CRA1 , the protein storage vacuole-localized membrane protein gene α-TIP , SSP processing enzyme gene δ-VPE and the ABA-responsive seed maturation gene At3g02480 , in wild type relative to the scl15-1 mutant seedlings ( Fig. 7d ), indicating that these genes are direct targets of HDA19–SCL15 interaction. ABI3 and Oleo2 did not show significant differences of HDA19 enrichment in the examined promoter regions between wild type and the scl15-1 mutant. The important phases of seed development are embryogenesis and seed maturation. The initiation and termination of the seed maturation phase and transition to germination and vegetative growth depend on the maintenance of cell fates and the correct deployment of developmental programmes. Many of the developmental processes active during seed maturation and seed filling are repressed after seed germination and seedling establishment. An increasing body of evidence has shown that chromatin remodelling is the key mechanism underlying repression of embryonic traits in vegetative tissues. The present work demonstrates a novel function for the GRAS family protein SCL15 in preventing the expression of embryonic traits during vegetative growth. SCL15 possesses conserved domains characteristic of the GRAS family of transcription factors. Localization of SCL15 to the nuclei of plant cells supports its role in transcriptional regulation of gene expression. SCL proteins are a major subfamily of the GRAS proteins, which comprise several groups. Thus far, only a few SCLs have been functionally characterized [31] , [36] , [37] , [38] . Three miR171 targets, namely SCL6/SCL6-IV, SCL22/SCL6-III and SCL27/SCL6-II (ref. 39 ), but also known as AtHAM3/LOM3, AtHAM2/LOM2 and AtHAM1/LOM1, respectively, were found to play a role in maintaining shoot meristem [28] , [40] . However, SCL6/AtHAM3 was also shown to be involved in the regulation of shoot branching [41] . Recently, SCL27/AtHAM1 was demonstrated to be involved in regulating chlorophyll biosynthesis via direct targeting G(A/G)(A/T)AA(A/T)GT cis -elements in the protochlorophyllide oxidoreductase gene [42] . SCL15 (also referred to as AtHAM4 ) was shown to be functionally redundant with AtHAM1 and AtHAM2 based on a secondary meristem phenotype in Atham1,4; Atham2/+ mutants [28] . Given the fact that SCL15 is not regulated by miR171, is evolutionarily divergent from AtHAM1 and AtHAM2 (ref. 28 ), and exhibits distinct cell type-specific expression patterns in Arabidopsis roots, we suggest that the role of SCL15 in promoting shoot indeterminacy is limited. Analysis of transcript levels of major embryonic genes and accumulation of SSPs in scl15 seedlings revealed that SCL15 plays an important role in controlling the embryonic phase to seedling transition through negative regulation of the seed-specific regulatory network. In other studies, several regulators, such as PKL, VALs and ASIL1, contribute to prevent ectopic expression of embryonic genes in seedlings [8] , [14] , [23] . It is noted that these transcriptional regulators may act to selectively repress certain embryonic genes, but not all. The key regulators LEC1 and ABI3 , the SSP genes CRA1 and CRU3 , and the major oleosin gene Oleo2 were substantially derepressed in scl15 seedlings. Transcript levels of δ- VPE , α-TIP and RTNLB13 , which are preferentially expressed in developing seeds and are essential for SSP trafficking and processing [35] , were dramatically elevated in scl15 vegetative tissues. This global gene expression profile in seedlings resembles that in developing seeds at the late phase of embryogenesis. Moreover, the seed storage protein 12S globulin accumulated in scl15 seedlings. Given the fact that scl15 mutant plants display no striking abnormalities in development or growth compared with wild type and that embryonic traits were derepressed in the mutant seedlings, we suggest that Arabidopsis plants can endure a certain level of seed-specific gene expression in vegetative tissues. Taken together, these results suggest that SCL15 mutation leads to a metabolic shift in vegetative tissues towards that of late embryogenesis and that SCL15 is required for the negative regulation of seed maturation genes in seedlings. Expression analysis has shown that regulators for repressing the seed maturation programme, such as PKL, VALs and ASIL1, are not only expressed in vegetative tissues, but also in the embryos of developing seeds [23] . In contrast, SCL15 is not expressed in the embryo, but is restricted to the vasculature of Arabidopsis leaves, roots, stems and siliques. SCL15 was localized in the phloem CCs and neighbouring tissues including leaf BS cells, root Pp cells and the placentochalaza region of the seed coat. This cell type-specific expression patterns leads to the speculation that, in addition to the CCs, the BS cells in leaves and the Pp cells in roots may be important sites for SCL15-regulated ectopic expression of embryonic traits in vegetative tissues. Although there is no direct evidence showing subcellular localization of seed storage reserves in vegetative tissues, the accumulation of vegetative storage proteins has been shown to be restricted to specialized cells including the vascular system in soybean stems, the BS cells in soybean leaves and the bark phloem tissues of trees [43] , [44] . Most HDACs are found to be part of large multiprotein complexes that are composed of transcriptional repressors and co-repressors [24] . HDAC-associated cofactors appear to be essential for the deacetylation of histones. It has been demonstrated that the specificity of HDAC-associated components impacts substrate selection and ultimately HDAC-mediated repression of target genes [45] . Trichostatin A inhibits HDAC activity during germination and results in elevated expression of embryogenesis-related genes. HDA19 is also known to prevent the expression of embryonic traits after seed germination and has been demonstrated to interact with VAL2 (refs 18 , 27 ); however, little is known about how this regulatory effect is exerted at a molecular level. In vitro and in planta protein–protein interaction assays indicate that SCL15 acts as a HDA19-associated regulator. Studies on the effect of scl15 mutation on histone acetylation at seed-specific genes and identification of some embryonic genes as direct targets of HDA19–SCL15 interaction indicate a functional association between SCL15 and HDAC in mediating repression of seed maturation genes in Arabidopsis seedlings. Given the contribution of HDA19 to embryonic gene repression after germination, our data suggest that ectopic expression of embryonic traits in scl15 mutant seedlings was due, at least in part, to increased histone acetylation levels at the seed-specific loci. SCL15 appears to interact with HDA19 to regulate the embryo-to-seedling phase transition. However, HDA6 was also shown to repress embryonic traits in vegetative tissues [27] , and not all of the seed maturation genes that were derepressed in the scl15 seedlings were identified as direct targets of HDA19–SCL15 interaction. This suggests that other HDACs and/or factors may also contribute to SCL15-associated repression of seed maturation genes. Plant materials and treatments Arabidopsis thaliana ecotype Col-0 was used as the wild-type plant. T-DNA insertion lines SALK_110871 ( scl15-1) and GK292A11 ( scl15-2 ) (NASC ID: N427947) [46] were obtained from the ABRC (Ohio State University) and the NASC (University of Nottingham), respectively. Arabidopsis plants were grown in pots of soil in a growth chamber that was set to 22 °C day/16 °C night on a 16/8 h day/night cycle and 60% relative humidity. Arabidopsis siliques were harvested at the heart to linear (5 DPA), mature (10 DPA) and post-mature (16 DPA) stages of embryo development. Seeds were completely dried after 17 DPA. To grow plants on solid medium, surface-sterilized seeds were kept for 2 days at 4 °C in the dark, placed onto 1/2 MS medium containing 0.7% agar and 1% sucrose, and grown at 22 °C under continuous light. Tobacco ( Nicotiana tabacum ) plants were cultivated in pots of soil in a growth chamber at 22 °C under long day conditions (16/8 h day/night). For ABA treatments, 14-day-old Arabidopsis seedlings were transferred from the 1/2 MS agar-sucrose plates to fresh plates containing the same medium with 0 or 50 μM ABA (A1049; Sigma-Aldrich) and harvested after incubation for 2 days. For the treatment with auxin, GA and sugar, 14-day-old seedlings were incubated in liquid half-strength MS medium supplemented with various concentrations of hormones or sucrose for 1 h. Mock (control) treatment consisted of no or 0.1% ethanol, as the IAA (I2886; Sigma-Aldrich) and GA 3 (G7645; Sigma-Aldrich) were dissolved in water and 0.1% ethanol, respectively. ChIP analysis was conducted using 3-week-old Arabidopsis seedlings grown on solid medium plates as described above. Roots of 14-day-old seedlings that were grown on solid medium and treated with 0 or 100 μM ABA (Sigma-Aldrich) for 4 h were used for co-IP assays. All tissues were harvested and flash frozen in liquid nitrogen and stored at −80 °C until used for RNA isolation and protein extraction. Identification of T-DNA insertion lines Individual plants from T-DNA-tagged lines were genotyped by PCR. The SCL15 -specific primers scl-f1 and scl-KO-r1 were used for identification of the wild-type allele and T-DNA left border-specific primer LBb1 and the SCL15 -specific primer scl-f1 were used to detect the mutant allele ( Supplementary Data 3 for all primer sequences). The position and structure of the T-DNA insertion site were analysed by PCR, Southern blotting and sequencing of the PCR products that spanned the insertion site. Individual homozygous plants were used for total RNA isolation, RT–PCR and real-time RT–PCR. Yeast two-hybrid screening For construction of the yeast two-hybrid cDNA library, total RNA was isolated from 2-week-old Arabidopsis seedlings, converted to cDNA and cloned into a GAL4 activation domain (GAL4 AD) vector pPC86. The SuperScript Plasmid System (Life Technologies) was used for cDNA synthesis and cloning. The open reading frame of the Arabidopsis HDA19 (Accession no. AY093153; At4g38130) was generated by PCR using primers HDA19-f1 and HDA19-r2, and cloned into the Sal I- Not I sites of pDBLeu in-frame with the GAL4 DB. This construct served as a bait to screen a cDNA library using the ProQuest Two-Hybrid System (Life Technologies) as previously described [47] . Candidate positive clones were confirmed by yeast retransformation and DNA sequencing analysis. 5′-RLM-RACE (Applied Biosystems/Ambion) was undertaken to determine the transcription start sites of candidate genes based on the manufacturer’s instructions. Alignment and phylogenetic analysis of amino-acid sequences Alignment of amino-acid sequences was performed using the AlignX programme, Vector NTI Advance 11 suite (Invitrogen), with default settings [48] . A neighbour-joining phylogenetic tree was generated using MEGA 5 (ref. 49 ) with default parameters. In vitro protein interaction assays The coding region of the Arabidopsis HDA 19 was amplified by PCR using HDA19-f2 and HDA19-r3 primers and inserted in-frame with GST into the Sal I and Not I sites of vector pGEX-6P-2 (Amersham Pharmacia). Expression, purification and western blotting analysis of the recombinant HDA19 was carried out as described by Gao et al. [50] . The entire coding region of SCL15 was amplified by PCR using scl-f3 and scl-r3 primers and cloned into the Hin dIII and Xho I sites of the expression vector pET-28b (Novagen) in-frame with the His-Tag sequence. The full-length SCL15 protein labelled with [ 35 S]methionine was produced using T N T–Quick Coupled Transcription/Translation System (Promega) according to the manufacturer’s instructions. In vitro protein interaction was detected using a GST pull-down assays as previously described [50] . Briefly, GST or GST-fusion protein was incubated with [ 35 S]Met-labelled translation mixture in a bead-binding buffer (50 mM K-phosphate (pH 7.6), 450 mM KCl, 10 mM MgCl 2 , 10% glycerol, 1% Triton X-100, 1% BSA and 1 μl per 50 ml of buffer of 1:12 diluted protease inhibitors set (Roche Diagnostics)). After incubation for 1 h at room temperature, a 50% slurry of glutathione-Sepharose beads containing 10 mg ml −1 of BSA and 4 μg of ethidium bromide was mixed with the interaction mixture followed by gentle rotation for 1 h at 4 °C. After washing six times with bead-binding buffer without BSA or ethidium bromide, but containing the protease inhibitors set, the bound proteins were eluted with 2 × SDS–polyacrylamide gel electrophoresis (PAGE) loading buffer and analysed by 12% SDS–PAGE. After electrophoresis, the gels were dried and subjected to fluorography. Full scans of the fluorographic films are provided in Supplementary Fig. 9 . BiFC assays DNA sequences for the N-terminal 173-amino-acid EYFP (N-YFP) and C-terminal 64-amino-acid (C-YFP) fragments were amplified previously by PCR and cloned into the plant expression vectors pOCA30 and pFGC5941 to generate pOCA-N-YFP and pFGC-C-YFP, respectively [51] . N-YFP was also cloned into pFGC5941 to generate a second N-YFP fusion/expression vector (pFGC-N-YFP). WRKY38 -coding sequence was amplified using primers WRKY38-f1 and WRKY38-r2, digested with Sac I/ Spe I and ligated into the Sac I- Xba I sites of pOCA-N-YFP to generate an in-frame fusion with N-YFP. The HDA19 -coding sequence was amplified using primers HDA19-f2 and HDA19-r3, digested with Spe I and Bg lII and ligated into the Xba I- Bam HI sites of pFGC-C-YFP to form an in-frame fusion with C-YFP. For generating the SCL15-N-YFP fusion construct, the ∼ 600 bp 5′ and ∼ 900 bp 3′ coding sequences of SCL15 were amplified using two pairs of primers scl-f6/scl-r6 and scl-f7/scl-r7, digested with Sac I/ Bam HI and Bam HI/ Xba I, respectively, and sequentially cloned into the same sites of pFGC-N-YFP. WRKY38 was sub-cloned in the same way as SCL15 and was used as a positive control for interaction with HDA19 (ref. 51 ). The plasmids were used for BiFC assays as previously described [52] . Fluorescence and Hoechst 33258 staining were visualized using a Zeiss LSM 710 confocal microscope. In the absence of Hoechst 33258 staining, fluorescence and chlorophyll were excited with YFP excitation and red channel, respectively, on a Zeiss Axio Imager Z1 microscope with ApoTome and AxioCam MRm (Carl Zeiss). The experiments were performed three times with the same results. Extraction of nuclear proteins and co-IP assays Nuclei and nuclear proteins were isolated from roots of 2-week-old Col-0 and SCL15pro::SCL15-sGFP (Compl-6) seedlings as previously described [53] . Briefly, root powder was homogenized in cold Buffer A (0.4 M sucrose, 10 mM HEPES, 2.5 mM dithiothreitol, 2 mM EDTA, 1 mM phenylmethylsulfonyl fluoride, 1 protease inhibitor cocktail tablet (Roche Diagnostics) per 50 ml buffer, pH 8). After filtration and centrifugation (14,000 g ) of the extracts, the pellet was resuspended in 1 ml of cold Buffer B (0.25 M sucrose, 10 mM HEPES, 1% Triton X-100, 10 mM MgCl 2 , 1 mM phenylmethylsulfonyl fluoride, protease inhibitor cocktail, pH 8) and centrifuged at 10,000 g for 10 min at 4 °C. The resultant pellet was resuspended in 300 μl of cold Buffer C (1.7 M sucrose, 10 mM HEPES, 0.15% Triton X-100, 2 mM MgCl 2 , 1 mM phenylmethylsulfonyl fluoride, protease inhibitor cocktail, pH 8). The pellet suspension was then carefully overlaid on top of 500 μl of Buffer C and centrifuged at 16,000 g for 45 min (4 °C). To release the nuclear proteins from the enriched nuclei, 300 μl of 1 × IP protein extraction buffer (100 mM NaCl, protease inhibitor cocktail, 110 mM KOAc and 0.5% Triton X-100, pH 7.4) was added to the cold nuclei suspension and subsequently sonicated with a sonicator (Qsonica, Model Q55) set at 35% amplitude for five times with 10 s for each sonication. After addition of 2 μl of benzonase (Sigma) to remove nucleic acids, the mixture was centrifuged at 12,000 g for 30 min at 4 °C and the proteins remaining in the supernatant were quantified. Co-IP assays were carried out with a kit using Dynabeads (Life Technologies) following the manufacturer’s instructions. Briefly, total nuclear proteins (300 μg) were pre-cleared with 1 mg of magnetic beads through continual rotation for 1 h at 4 °C. Polyclonal anti-GFP antibody (7.5 μg; Clontech, Catalogue No. 632592) was coupled to 1.5 mg of magnetic beads at a dilution of 1:200 following the manufacturer’s instructions and then incubated with the pre-cleared nuclear protein extract by rotating for 30 min at 4 °C. The immobilized proteins on the GFP-coupled beads were washed four times and subsequently eluted for immunoblotting using anti-HDA19 antibodies [54] at a dilution of 1:2,000 and HRP-conjugated goat anti-rabbit IgG (Invitrogen, Catalogue No. 65–6120) as the secondary antibody at 1:30,000 dilution. The Clarity Western ECL Substrate system (Bio-Rad) was used for immunodetection of HDA19. Full scans of the western blots are shown in Supplementary Fig. 10 . ChIP assays in yeast The effector plasmid SCL15-GAL4BD was constructed by ligating the amplified SCL15 product (primers scl-f4 and scl-r4) between the Sal I and Not I sites of the vector pDBLeu (Life Technologies) in-frame with the GAL4BD sequence. To make the construct p426GAL1-HAD19 , plasmid pDBLeu-HDA19 was digested with Sal I and Not I and the HDA19 fragment cloned between the Sal I and Not I sites of the vector p426 GAL1 (Life Technologies). MaV203 yeast cells, expressing an integrated lac Z reporter gene driven by the GAL1 promoter ( GAL1pro ; Life Technologies), were transformed with either the effector SCL15-GAL4BD only, both SCL15-GAL4BD and p426GAL1-HDA19 , or empty vectors pDBLeu and p426 GAL1 . The β-galactosidase activity was measured using chlorophenol red-β- D -galactopyranoside. Quantitative data (mean±s.d.) were determined from three independent assays. The GAL1pro contains distant GAL4BD sites located in the 365-bp upstream activation sequence UAS G designated as UAS GAL1 (ref. 55 ). ChIP experiments were performed as previously reported [47] using anti-acetyl-histone H3K9 antibody (07–352; Millipore). DNA enrichment was analysed by real-time quantitative PCR (qPCR) using specific primers. Three replicates of the ChIP assay were carried out on different preparations of nuclei. ChIP assays in Arabidopsis ChIP experiment was conducted as described previously [56] . Chromatin extract was prepared from seedlings treated with formaldehyde. After being sheared to an average length of 500 bp by sonication, the chromatin was immunoprecipitated with specific antibodies, including anti-acetyl-histone H3K9K14 (06–599; Millipore), anti-acetyl-histone H4K5K8K12K16 (06–866; Millipore) and anti-HDA19 (ref. 54 ). qPCR was carried out to detect the DNA cross-linked to the immunoprecipitated proteins. Primers used for qPCR analysis in ChIP assays were designed within 350 bp around the transcription initiation sites (promoter region) or to flank the ATG translation start site (ATG region; Supplementary Fig. 8 ). Primer sequences are given in Supplementary Data 3 . ACT7 was used as internal control for normalization [7] . Each immunoprecipitation was replicated a minimum of three times and each sample was quantified in triplicate. All results were shown as means±s.d. of at least three biological replicates. Plasmid construction For subcellular protein localization, the construct 35Spro::smRS-GFP was generated in the binary vector pCAMBIA [57] by subcloning the cDNA (U70496) that encodes the smRS-GFP [58] . The SCL15 open reading frame was amplified by PCR and subcloned into the EcoR I- Sac II sites of the plasmid 35Spro::smRS-GFP in-frame with the N-terminus of smRS-GFP generating 35Spro::SCL15-smRS-GFP . Plasmid 35Spro::smRS-GFP was used as the negative control for transient expression in Nicotiana tabacum epidermal cells [59] . For promoter expression studies, 2,353 bp of the SCL15 promoter including 299 bp of 5′ untranslated region was amplified using primer pairs scl-f8 and scl-r8 and cloned into the binary vector pBI121 by replacing the CaMV 35S promoter. The SCL15pro::GUS plasmid was introduced into Agrobacterium tumefaciens strain GV3101 followed by transformation into Arabidopsis plants using the floral dipping method [60] . For complementation of the scl15 mutant, the SCL15 gene sequence (including 2,051 bp of promoter, the 5′ untranslated region and 1,458 bp of coding region without the TAG stop codon) was synthesized in frame with 717 bp of sGFP by GeneArt Gene Synthesis (Life Technologies, Canada), in which a ten-residue flexible polypeptide linker (GGGGSGGGGS) was inserted before sGFP , and cloned into a modified pZP121 binary vector [57] . The resulting SCL15pro::SCL15-sGFP construct was used to transform homozygous scl15-1 mutant plants. Multiple independent transgenic lines that displayed a 3:1 segregation ratio in T2 populations were selected. The T3 homozygous lines Compl-6 and Compl-8 were chosen for the complementation assays. Histochemical and microscopic analysis For subcellular localization of the SCL15:smRS-GFP fusion, transiently transformed N. tabacum leaves were incubated with 50 μg ml −1 4',6-diamidino-2-phenylindole (DAPI; Life Technologies) for nuclei staining. Leaf tissues were stained with DAPI for 30 min. GFP signal was observed on a Zeiss Axio Imager Z1 microscope with ApoTome and AxioCam MRm and AxioVision Rel. 4.7 Imaging System (Carl Zeiss) with excitation of 490 and 383 nm for GFP and DAPI, respectively. The images shown are representative of at least three independent experiments. For SCL15pro::GUS activity assay, whole Arabidopsis seedlings or individual organs were incubated with GUS staining solution (10 mM phosphate buffer, 10 mM EDTA, 0.1% (v/v) Triton X-100, 1 mM potassium ferricyanide, 1 mM potassium ferrocyanide, 1 mg per 1 ml of X-Gluc (5-bromo-4-chloro-3-indolyl-β-D-glucuronide) from 50 mg ml −1 stock in dimethylformamide). Samples were mounted in water under a coverslip and viewed using a Zeiss Axio Imager Z1 microscope. For histological analysis of transverse sections of Arabidopsis tissues, GUS staining was performed as described by Sieburth and Meyerowitz [61] . Images were captured using an Axioplan Universal microscope with a Digital CCD camera and AxioCam ICc 1 and AxioVision Release 4.7 software. For anatomical analysis of SCL15pro::SCL15-sGFP plants, whole seedlings were stained briefly with 10 μg ml −1 propidium iodide (Sigma-Aldrich), mounted in water under glass coverslips, and visualized on a Zeiss Axio Imager Z1 microscope with ApoTome and AxioCam MRm software. The excitation wavelengths for GFP and propidium iodide were 561 nm and 488 nm, respectively. Microarray and data analysis Wild-type Col-0 and scl15-1 seeds were sterilized and sown onto 1/2 MS agar-sucrose plates. Total RNA was isolated from 14-day-old seedlings using the RNeasy Plant mini kit (Qiagen). An Arabidopsis 70-mer oligo-gene array containing 26,090 annotated genes was used for microarray analysis. The GeneChip arrays were developed by Qiagen/Operon and printed on Super Amine slides (Telechem International) at the Microarray and Proteomics Facility, University of Alberta, Edmonton, AB, Canada. Total RNA was amplified and probe was labelled using an Ambion Amino Allyl MessageAmp II RNA amplification kit (Ambion) according to the manufacturer’s instructions as described previously [62] . Total RNA from three independent biological replicates were used. Briefly, fluorescent cDNA probes were synthesized from RNA and labelled with Cy3- or Cy5-dCTP using CyDye Post-Labelling Reactive Dye Packs (GE Healthcare). Hybridization and washing were performed according to the Corning Epoxide Coated Slides instruction manual (Corning Life Sciences). The labelled antisense RNA was fragmented in Ambion's fragmentation buffer (Applied Biosystems). After addition of 45 μl of DIG Easy Hybridization solution (Roche, Diagnostics) and 3 μl of blocking buffer (GE Healthcare) followed by incubation for 2 min at 65 °C, samples were hybridized for 16–18 h at 37 °C using a MAUI hybridization system (BioMicro Systems). Microarray images were analysed using Array-Pro Analyzer software (Media Cybernetics). The data were then extracted, log transformed, quantile normalized and corrected for background using Robust Multiarray Analysis. Statistical analysis of gene expression data was based on the Student’s t -test ( P ≤0.05) and a Benjamini-Hochberg false discovery rate multiple testing correction with cutoff of 0.05 (ref. 63 ). Differentially expressed genes were considered to be those exhibiting at least a twofold change. GO categories that were significantly over-represented among upregulated genes in the scl15-1 seedlings were determined using the Biological Network Gene Ontology tool 2.4 (BiNGO 2.4) plugin [34] for Cytoscape 2.8 (ref. 64 ) with default settings (hypergeometric test and a Benjamini-Hochberg multiple testing correction [63] ). qRT–PCR analysis Total RNA was extracted from Arabidopsis seedlings or siliques using the RNeasy Plant Mini Kit (Qiagen) and genomic DNA was eliminated from RNA samples with DNase I (amplilification grade; Life Technologies). Total RNA was reversed transcribed using the SuperScript III First-Strand Synthesis SuperMix for qRT–PCR (Life Technologies) following the manufacturer’s instructions. Real-time RT–PCR was performed using the Platinum SYBR Green qPCR SuperMix-UDG (Life Technologies) on an ABI Prism StepOnePlus Real-time PCR System (Applied Biosystems) or using the SsoFast EvaGreen Supermix (Bio-Rad) in a CFX96 Touch Real-Time PCR Detection System (Bio-Rad) according to the manufacturer’s instructions. ACT2 and Ef-1α were used as the reference genes. Each pair of primers produced a single amplicon of the expected size and melting temperature. The gene-specific primers for LEC1 , ABI3 , CRU3 , RAB18 , Oleo2 , Ef-1α and ACT2 have been described previously [23] and those for other genes are listed in Supplementary Data 3 . Data were analysed using the StepOne Software v2.0 (Applied Biosystems) or the CFX Manager 3.1 (Bio-Rad). All samples were run with triplicate and results present are the mean (±s.d.) of three biological replicates. Immunoblotting Arabidopsis 12S globulin was purified by HPLC and a monoclonal anti-12S globulin CRA1 was generated by the Animal Care Unit, Western College of Veterinary Medicine, University of Saskatchewan, Saskatoon, Canada. 12S globulin were purified from leaves of 2-week-old Col-0 and scl15-1 plants following treatment with or without 50 μM ABA for 2 days by employing a RuBisCO depletion and antibody-capture technique. Briefly, 100 μg of ground leaf tissues was combined with 500 μl protein extraction buffer (7 M urea, 2 M thiourea, 50 mM Tris-HCl, pH 9.0, 0.2% Triton X-100, one Complete Protease Inhibitor Cocktail Tablet (Roche Diagnostics) per 30 ml). Following homogenization with a micropestle and centrifugation at 7,800 g at 4 °C for 20 min, supernatants were clarified by passage through a 0.45-μm syringe filter and centrifugation at 10,000 g , 4 °C for 1 min. For each supernatant, 500 μg protein was subjected to Rubisco depletion using Seppro Rubisco Spin Columns (Sigma-Aldrich) and then used directly for antibody capture using rabbit anti-globulin polyclonal-coupled Dynabeads Protein G (Life Technologies) according to the manufacturer’s instructions. Enriched 12S globulin species were eluted, boiled and resolved by 15% SDS–PAGE for silver staining and immunoblotting analysis. For detection of globulin species, a 1:1,000 dilution of monoclonal anti-CRA1 antibody and a 1:5,000 dilution of anti-mouse-HRP (Bio-Rad,Catalogue #170–6516) were employed along with Immobilon Western Chemiluminescence HRP Substrate (Millipore) according to the manufacturer’s instructions. A full scan of the immunoblot is presented in Supplementary Fig. 11 . Accession codes: The microarray data were deposited to NCBI Gene Expression Omnibus under the accession code GSE67395 . How to cite this article: Gao, M.-J. et al. SCARECROW-LIKE15 interacts with HISTONE DEACETYLASE19 and is essential for repressing the seed maturation programme. Nat. Commun. 6:7243 doi: 10.1038/ncomms8243 (2015).